Breeding latitude drives individual schedules in a trans-hemispheric migrant bird Despite clear benefits of optimal arrival time on breeding grounds, migration schedules may vary with an individual bird's innate quality, non-breeding habitat or breeding destination. Here, we show that for the bar-tailed godwit ( Limosa lapponica baueri ), a shorebird that makes the longest known non-stop migratory flights of any bird, timing of migration for individual birds from a non-breeding site in New Zealand was strongly correlated with their specific breeding latitudes in Alaska, USA, a 16,000–18,000 km journey away. Furthermore, this variation carried over even to the southbound return migration, 6 months later, with birds returning to New Zealand in approximately the same order in which they departed. These tightly scheduled movements on a global scale suggest endogenously controlled routines, with breeding site as the primary driver of temporal variation throughout the annual cycle. Some migratory birds 'winter' vast distances from where they nest, yet are under strong selection pressure to arrive on the breeding grounds at the time that best assures successful reproduction. Despite clear links between the timing and success of breeding, substantial variation exists in the migration timing of individual birds, which can largely be explained in terms of three primary mechanisms: (1) variation in individual quality; (2) variation in fuelling resources; and (3) geographical variation among breeding destinations. In the first case, which has received the most attention in studies of migration timing, birds possess heritable or acquired differences in moulting or fuelling efficiency, with only the highest-quality birds achieving an optimal migration schedule [1] . In the second, birds from high-quality non-breeding habitats may migrate earlier than those in low-quality habitats [2] , [3] and consequently experience increased breeding success [4] . The third scenario involves geographical variation in temporal availability of breeding resources, resulting in individual birds having different optimal schedules based on their respective breeding sites. This phenomenon is easily illustrated when races of the same species have clear differences in breeding range and migration timing [5] , [6] , but within-population demonstrations are rare. For example, tundra-breeding birds at northerly latitudes generally begin nesting as soon as snow recedes from their breeding sites [7] . Within Alaska, tundra becomes snow-free 2–4 weeks earlier in the southwest than it does in the far north [8] . As a result, optimal arrival dates for birds in widely distributed breeding populations may vary substantially [9] . Bar-tailed godwits ( Limosa lapponica baueri ) depart New Zealand during March and early April, and fly ~10,000 km to sites on the Yellow Sea coast of Korea and China [10] . After refuelling, godwits depart Asia from late April to late May, and fly ~6,000 km to coastal sites in southwestern Alaska. They then disperse to coastal tundra sites across western and northern Alaska (59–71° N latitude) for breeding in May–July. The godwits then congregate in southwestern Alaska to refuel before departing in late August–early October on a non-stop trans-Pacific flight of 11,000–12,000 km to New Zealand, the longest non-stop flight recorded in birds [11] . The difficulty of tracking small-bodied birds across great distances has hampered our understanding of cross-seasonal interactions between events on opposite sides of the globe. Studies are often limited to methods (for example, stable isotopes) that require indirect steps to link the breeding and non-breeding grounds of individual birds. The advent of small, lightweight geolocators allows these links to be made directly [12] , but the need to retrieve units to access data has limited their use to site-faithful species using accessible, high-density breeding sites [13] , [14] . Bar-tailed godwits breed cryptically in low densities across over 1,800 km of remote coastal tundra within Alaska [10] , making breeding studies extremely difficult. However, high non-breeding site fidelity of godwits in New Zealand allows the use of geolocators for inferences across the entire breeding range, while controlling for non-breeding habitat quality. Our study is the first to deploy geolocators on non-breeding birds, and also the first involving shorebirds (suborder Charadrii), a group famous for extreme long-distance migrations. We attached geolocators to non-breeding bar-tailed godwits at a small estuary in New Zealand, and recaptured them after their return migration. We show that the timing of each step in a >30,000 km round-trip migration (northbound departure from New Zealand, departure from fuelling sites in Asia, arrival on Alaskan breeding grounds and subsequent southbound departure) is primarily dependent on the latitude of an individual bird's breeding site. Timing of migration Godwits ( Fig. 1 ) from our study site used breeding sites spanning 59.7–70.2° N latitude ( Fig. 2 ), encompassing most of the known Alaskan breeding range for the subspecies. Northerly breeders migrated later than southerly breeders in each phase of the northward journey: departure date from New Zealand was significantly correlated with breeding latitude ( Fig. 3a ), as were Yellow Sea departure ( Fig. 3b ) and date of arrival at breeding sites ( Fig. 3c ). The correlation between New Zealand departure date and the location of a breeding site a 16,000–18,000 km journey away, strongly suggests endogenously controlled schedules, as environmental cues indicating tundra conditions in the opposite hemisphere are improbable. The relationship between migration timing and latitude became stronger with each stage of the northbound migration, implying a tightening of these programmed schedules with proximity to the breeding grounds. For the postbreeding southbound return flight, northerly breeders again migrated later: departure date from Alaska was significantly correlated with breeding latitude ( Fig. 3d ). 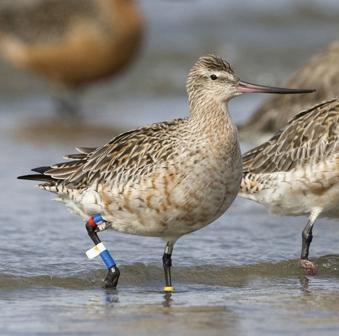Figure 1: Light-sensitive geolocator. Individually colour-banded male bar-tailed godwit with tibia-mounted geolocator, before departure from New Zealand. Photo by Phil Battley. Figure 1: Light-sensitive geolocator. Individually colour-banded male bar-tailed godwit with tibia-mounted geolocator, before departure from New Zealand. Photo by Phil Battley. 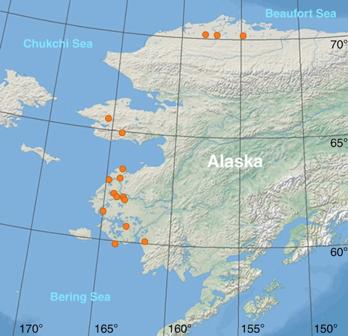Figure 2: Alaskan breeding locations. Breeding locations derived from geolocators for 16 bar-tailed godwits tracked from New Zealand. Full size image Figure 2: Alaskan breeding locations. Breeding locations derived from geolocators for 16 bar-tailed godwits tracked from New Zealand. 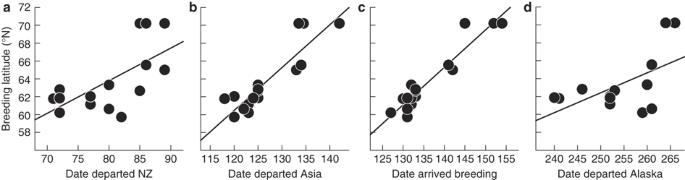Figure 3: Breeding latitude and timing of migration. Timing of migration of bar-tailed godwits was correlated with breeding latitude in Alaska. Some overlapping points have been neutrally offset for clarity. Figure axes have been transposed to aid visualization of geographical relationships. (a) Date (day 1=1 January) of departure from New Zealand in relation to breeding latitude (r2=0.45, slope=1.22 ± 0.36,n=16,P=0.005). (b) Date of departure from the Yellow Sea in relation to breeding latitude (r2=0.80, slope=1.67 ± 0.22,n=16,P<0.001). (c) Date of arrival on breeding grounds in relation to breeding latitude (r2=0.91, slope=2.16 ± 0.19,n=16,P<0.001). (d) Date of departure from Alaska in relation to breeding latitude (r2=0.32, slope=1.43 ± 0.64,n=13,P=0.046). Full size image Figure 3: Breeding latitude and timing of migration. Timing of migration of bar-tailed godwits was correlated with breeding latitude in Alaska. Some overlapping points have been neutrally offset for clarity. Figure axes have been transposed to aid visualization of geographical relationships. ( a ) Date (day 1=1 January) of departure from New Zealand in relation to breeding latitude ( r 2 =0.45, slope=1.22 ± 0.36, n =16, P =0.005). ( b ) Date of departure from the Yellow Sea in relation to breeding latitude ( r 2 =0.80, slope=1.67 ± 0.22, n =16, P <0.001). ( c ) Date of arrival on breeding grounds in relation to breeding latitude ( r 2 =0.91, slope=2.16 ± 0.19, n =16, P <0.001). ( d ) Date of departure from Alaska in relation to breeding latitude ( r 2 =0.32, slope=1.43 ± 0.64, n =13, P =0.046). Full size image Duration of stopover in the Yellow Sea was highly variable (30–50 days), which may reflect individual strategies with regard to moult and fuelling, or variation in stopover site quality. Godwits use fuelling sites spanning 600 km of latitude in the Yellow Sea, and these sites vary significantly in size, level of human impacts and competition with other migrating shorebirds. There was no apparent relationship between the choice of fuelling site and timing of migration, stopover duration or breeding latitude. However, stopover duration for godwits breeding at higher latitudes was greater than those breeding farther south ( Fig. 4 ). Similarly, after arrival in Alaska, northerly breeders remained at coastal sites slightly longer before moving to breeding sites (range: 0–13 days; duration versus breeding latitude: r 2 =0.32, n =16, P =0.023). Thus, the variation among individual birds increased with each successive segment of the migration (range of New Zealand departure=20 days; Yellow Sea departure=23 days; breeding arrival=28 days), and total travel time from New Zealand to breeding sites increased with breeding latitude (range: 48–67 days; duration versus breeding latitude: r 2 =0.40, n =16, P =0.009). This is unsurprising, as godwits breeding in northern Alaska must travel 1,000–1,600 km further than southerly breeders, and may require greater reserves to prepare for colder and less predictable conditions on their breeding grounds. 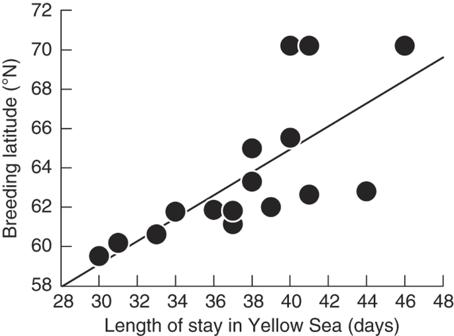Figure 4: Breeding latitude and stopover duration. Length of stay in the Yellow Sea for bar-tailed godwits on northbound migration was positively correlated with breeding latitude in Alaska (r2=0.51,n=16,P=0.002). Figure 4: Breeding latitude and stopover duration. Length of stay in the Yellow Sea for bar-tailed godwits on northbound migration was positively correlated with breeding latitude in Alaska ( r 2 =0.51, n =16, P =0.002). Full size image Although breeding arrival has well-understood time constraints, migration to non-breeding grounds is considered to be much less time-dependent [15] , [16] . However, birds departed Alaska in approximately the same order in which they departed New Zealand ( Fig. 5 ), and the span of departures from Alaska was 27 days, similar to the northbound migration. Breeding success creates great potential variation in the date that an individual bird may begin fuelling for southbound migration, because birds caring for young through fledging may invest 3–6 weeks more than those that fail during incubation. However, there was no evidence that failed breeders used this 'advantage' to achieve earlier southbound departure: total time spent in Alaska was nearly identical for successful (mean=125.0 days, n =4) and failed (mean=125.6 days, n =7) breeders. Furthermore, southerly breeders might be expected to migrate south later, because apparently suitable breeding conditions persist later at lower latitudes and offer greater renesting opportunity; our findings do not support this. These data suggest rigidity in the migration schedule, perhaps evolved to best exploit a predictable peak of fuelling resources or favourable wind conditions [5] necessary for the southbound flight. 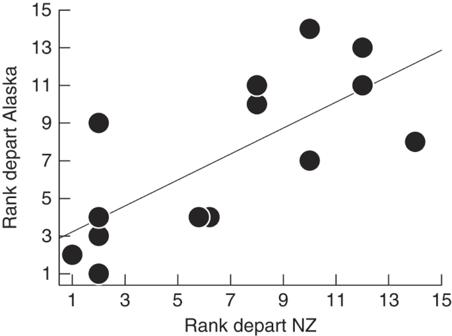Figure 5: Order of departure on northbound and southbound migration. Order of migratory departure from New Zealand and Alaska was similar for individual bar-tailed godwits (Spearman rank correlation:rs=0.74,n=14,P=0.003). Some overlapping points have been neutrally offset for clarity. Figure 5: Order of departure on northbound and southbound migration. Order of migratory departure from New Zealand and Alaska was similar for individual bar-tailed godwits (Spearman rank correlation: r s =0.74, n =14, P =0.003). Some overlapping points have been neutrally offset for clarity. Full size image Breeding plumage For species in which one sex competes for breeding partners or territories, variation in plumage may communicate relative individual quality to competitors or potential mates [17] . The extremely variable breeding plumage of male godwits has led to the hypothesis that redder males may be of higher quality, and therefore may migrate earlier than paler males [18] . In our study, the extent of male breeding plumage was unrelated to departure from New Zealand ( r 2 =0.36, n =9, P =0.87); this was also true at another non-breeding site in New Zealand [19] . However, redder males departed from the Yellow Sea later than paler males ( r 2 =0.46, n =9, P =0.044) and arrived later on the breeding grounds ( r 2 =0.79, n =7, P =0.007), contrary to the prediction, but similar to observations of L. l. taymyrensis in Europe [18] . Although supported in other species, the use of breeding plumage as an index of individual quality in bar-tailed godwits is far from straightforward. First, there is no empirical evidence linking breeding plumage with reproductive success in this species, and links with other parameters such as body condition, parasite loads or survival are equivocal [18] , [20] , [21] , [22] , [23] . Second, plumage varies geographically among Alaskan godwits, with redder males breeding at higher latitudes, on an average (J.R.C. and P.F.B., unpublished). Accordingly, redder males in this study bred at higher latitudes ( r 2 =0.73, n =7, P =0.015). However, because of continued contour moult during northbound stopover [21] , the degree of which may vary among individual birds, it is unknown how closely variation in plumage on New Zealand departure reflects that on the breeding grounds. Our findings implicate individually optimized breeding arrival date as the primary driver of variation in the migration schedule of godwits: latitude of an individual bird's breeding site (and, by extension, the approximate timing of snow melt from that patch of Alaskan tundra) could be traced back to that bird's departure from New Zealand 7–10 weeks earlier and more than half a world away. This strongly suggests endogenous programming of migration, and warns against quality-based inferences regarding any single stage of the migration without knowledge of the entire annual cycle. Nevertheless, competition and individual quality may yet function at a fine scale; that is, birds at the same latitude vary in quality, arrival date and breeding success. Our sample is insufficient to evaluate timing differences among birds breeding at the same latitude, but the small amount of variation in breeding arrival left unexplained by latitude itself (10%) suggests that such variation is relatively minor. Latitude is a coarse index for the earliest availability of a site, and does not account for small-scale geographical variation, which may promote differing optimal arrival dates even for sites at similar latitudes [7] . This makes the extremely tight relationship between breeding arrival and latitude all the more surprising. However, given the brief breeding season at high latitudes, it is nevertheless conceivable that a few days difference in arrival could significantly affect mate acquisition or retention [24] , or breeding success. If individual quality or condition were largely driving the timing of migration, we would expect early-arriving birds to maximize their reproductive potential by occupying the highest-quality breeding sites. Low-latitude breeding sites could be more desirable, because of a shorter migration distance, milder and more predictable conditions and a longer snow-free season. However, the drawbacks of breeding farther north may be offset by a latitudinal cline in nest predation rates [25] . Given the low breeding density of bar-tailed godwits and a general lack of evidence of food or habitat limitation among tundra-breeding shorebirds, it is improbable that early-arriving birds, through early occupation of low-latitude breeding sites, force later birds to breed at high latitudes. It is more likely that migration timing and breeding site are linked and heritable, and maintained by either genetic structure within the population or by environmentally mediated regulation of gene expression [26] . Some Holarctic shorebird species seem to have radiated across vast regions very recently, such that clear population differences in breeding range and migration are only weakly reflected in the genetic structure within the population [27] . In some cases, epigenetics, a field of vast potential for ecologists, may be the key mechanism for persistent intraspecific variation. Our study sheds light on results from previous bar-tailed godwit studies. At the Firth of Thames, New Zealand, individual godwits showed high annual repeatability of both the departure date and the extent of breeding plumage, but did not conform to expectations of 'high-quality' (redder) birds migrating earlier [19] . Similarly, male godwits, whose moult and mass indicated readiness for early departure, were paler and larger than males not yet in migratory condition [20] . Both of these results are now explained by the links between breeding site, timing and plumage. The similar later northbound departure of redder males in the European population ( L. l. taymyrensis ) [18] suggests that these patterns may exist across the entire range of the species, but that study found no evidence of geographical variation in plumage within the breeding range. Interestingly, the population structure within Alaska does not seem to persist in the non-breeding season. Other sites in New Zealand show a range of northbound departure dates similar to our study site [19] , [28] , suggesting that godwits from the entire Alaskan breeding range mix freely in the non-breeding season. For long-distance migrants, selection for the timing of breeding may occur at very different temporal and spatial scales than selection for timing of migration per se . In bar-tailed godwits, timing of migration seems quite consistent, both at the population and individual [19] level, despite substantial annual variation in the date of snow melt; this pattern seems to be common among tundra-breeding, long-distance migrant shorebirds [7] , [29] . Timing of long-distance flights likely evolved in response to long-term global patterns in the timing of fuelling resources and beneficial prevailing winds, whereas nesting phenology seems very sensitive to local and annual variation in conditions dictating the availability of breeding sites [7] . This may explain why timing of southbound migration was unresponsive to the apparent duration of breeding investment in our study. Unfortunately, the potentially conflicting pressures of optimal timing of migration and breeding may make long-distance migrants such as godwits particularly vulnerable to the effects of climate change [30] , if rigid flight schedules contribute to a mismatch between breeding arrival and optimal nest initiation [31] , or preclude adaptation to temporal shifts in resources or weather during migration. The departure of birds from New Zealand and Alaska (two events separated by 6 months and over 11,000 km) in approximately the same order and span of days is quite surprising, in light of potential intervening variation caused by individual differences in flight speed, stopover duration, migration distance, duration of suitable breeding conditions, breeding success, body size, moult speed, foraging ability and habitat quality. This relationship between timing of northbound and southbound migration, which lacks a clear theoretical foundation in migration literature [16] , may reflect constraints operating on the entire annual cycle. Although flexibility in duration and investment in annual activities such as moult [32] , [33] and fuelling [34] , and even in migration route [35] , have been demonstrated in other species, the extreme nature of the godwit's migration may naturally ensure reduced variation in these parameters. Accordingly, the specificity with which breeding site dictates migration timing and the rigid repeatability of individual migration schedules [19] seem especially high, compared with those found in shorter-distance migrant birds. Every New Zealand bar-tailed godwit breeding in Alaska must be capable of a 10,000 km non-stop flight to Asia, followed by a 6,000 km flight across the northern Pacific Ocean; this is surely among the most challenging migrations in birds. Low-quality birds are unlikely to complete this migration, and those in poor condition may not attempt it at all. It is unlikely that any truly 'low-quality' godwits reach the breeding grounds. This model of godwit migration suggests that a bird's breeding site is endogenously controlled, and all other annual events are shifted temporally to optimize arrival on the breeding grounds. Among the consequent predictions is that northerly breeders should exhibit delayed completion of feather moult and premigratory mass gain in New Zealand, and the duration of these activities may be relatively constant, regardless of migration schedule. Using migration timing as a reliable index for breeding latitude, these predictions are now testable by godwit studies restricted to non-breeding sites. We might also expect to find similar patterns in other long-distance migrant species in which birds from one non-breeding site may breed across vast geographical ranges (for example, great knots, Calidris tenuirostris [36] ). Geolocation data During two non-breeding seasons (2007–2008 and 2008–2009), we captured godwits from a small (200–280 birds) population at the Manawatu River estuary, New Zealand (40.47° S, 175.22° E) and attached leg-mounted [37] light-sensitive geolocators (British Antarctic Survey, model MK14; 1.4 g; 2-year life). The return rate of these birds was 95%; we recaptured 80% of those available. Some birds carried geolocators for two migrations, and some units failed during deployment; for each bird, we used the first year with the most complete data. We calculated breeding locations for 16 birds (7 males, 9 females); for 3 of these, the subsequent date of Alaska departure was unavailable because of geolocator failure. One other female was tracked for the entire migration, but did not settle at a breeding site (thus, n =14 in Fig. 5 ). The geolocators record sunrise/sunset, allowing the calculation of latitude and longitude (±130 km error, based on ground-truthing units and resightings of instrumented godwits), except during ±15 days of the vernal or autumnal equinox, when only longitude is reliable. To derive fuelling sites in Asia and breeding sites in Alaska, we averaged twice-daily locations over periods when birds were relatively stationary, excluding clear outliers caused by weather or bird behaviour. For three birds breeding north of the Arctic circle (thus providing no sunrise/sunset data during this time), we assumed a breeding latitude of 70.2° N (the known breeding range in this region occurs 69.5–70.8° N [10] ).On the basis of resightings of colour-marked godwits at the Manawatu River estuary, timing of migration was similar between years; mean northbound departure ( n =48 birds) and southbound arrival ( n =45 birds) in 2008 and 2009 differed by 0.48 and 1.0 days, respectively. In addition, snow-free dates for Alaskan breeding sites differed by <5 days between the 2 years [8] , despite annual variation of up to 18 days (1998–2009). Therefore, we combined geolocator data from 2008 (11 birds) and 2009 (6 birds) for analysis. Departure from the Manawatu River estuary was similar for colour-banded males and females in both years (2008: t 61 =1.42, P =0.16; 2009: t 60 =0.747, P =0.46), as was postbreeding return to the site (2008: t 51 =0.546, P =0.59; 2009: t 57 =0.807, P =0.42). Among geolocators, there was no apparent difference in migration timing between males and females after controlling for breeding latitude, although sample sizes were quite small. In addition, field observations on the breeding grounds provide no evidence for protandry in breeding arrival (J.R.C., personal observation). Therefore, we combined male and female geolocator data for analysis. Hatching success Geolocators also allowed estimation of hatching success by indicating periods of nest incubation [13] . During the breeding season, geolocators registered nights as regular, cleanly demarcated periods of 0–4.5 h of darkness, depending on latitude. Conversely, days appeared as continuous light, irregularly broken by very brief (<1 h) shading events, most likely corresponding to behaviours such as wading or sitting. Within 6–25 days of apparent arrival on breeding grounds, most birds displayed a conspicuous pattern of incubation, in which semiregular shading events of 4–13 h were overlayed on the day/night pattern for periods up to 25 days. When data clearly indicated incubation ( n =14), we designated birds as 'successful' (21–25 consecutive days of incubation; expected incubation duration 20–21 days [10] ) or 'failed' (<18 days). Breeding plumage Before departure from New Zealand, bar-tailed godwits undergo a breeding plumage moult, during which some portion of non-breeding ventral contour feathers is replaced with bold rufous-coloured feathers [10] . Using field observations and digital photographs, we scored breast and belly plumage on a scale of 1–7 [21] (1=no red feathers; 7=completely replaced with red feathers). Males carrying geolocators departed the study site with plumage scores of 4.5–5.5. Fieldwork was conducted with the Massey University Animal Ethics Committee approval (#07/163). How to cite this article: Conklin, J.R. et al . Breeding latitude drives individual schedules in a trans-hemispheric migrant bird. Nat. Commun. 1:67 doi: 10.1038/1072 (2010).